All optical reconfiguration of optomechanical filters Reconfigurable optical filters are of great importance for applications in optical communication and information processing. Of particular interest are tuning techniques that take advantage of mechanical deformation of the devices, as they offer wider tuning range. Here we demonstrate reconfiguration of coupled photonic crystal nanobeam cavities by using optical gradient force induced mechanical actuation. Propagating waveguide modes that exist over a wide wavelength range are used to actuate the structures and control the resonance of localized cavity modes. Using this all-optical approach, more than 18 linewidths of tuning range is demonstrated. Using an on-chip temperature self-referencing method, we determine that 20% of the total tuning was due to optomechanical reconfiguration and the rest due to thermo-optic effects. By operating the device at frequencies higher than the thermal cutoff, we show high-speed operation dominated by just optomechanical effects. Independent control of mechanical and optical resonances of our structures is also demonstrated. The combination of advances in the fields of nanomechanics and nanophotonics has resulted in the recent emergence of the field of nanoscale optomechanical (OM) systems [1] , [2] , [3] , [4] , [5] , [6] , [7] , [8] , [9] , opening the door to revolutionary capabilities [1] , [4] , [5] , [10] , [11] . Photonic crystal nanobeam cavities (PCNCs) [12] , [13] , [14] , [15] , [16] are well suited for the realization of OM systems due to their small footprint, wavelength scale and high-quality factor (Q) optical modes, small mass and flexibility. These features allow for manipulation of optical signals as well as mechanical properties of PCNCs at low powers [17] , a property that is of interest for dynamic signal filtering [18] , routing and modulation [19] . Here we discuss a fully integrated, reconfigurable optical filter that can be programmed using internal optical forces. The fundamental building block of our platform is a doubly clamped nanobeam mechanical resonator that is patterned with a one-dimensional lattice of holes to form a high-Q optical nanocavity [15] . When two such resonators are placed in close proximity their optical modes couple, resulting in sharp, wavelength-scale, optical resonances, which can be highly sensitive to the separation between the nanobeams [1] , [17] , [20] . In addition, the structure supports propagating waveguide modes that can be excited over a wide wavelength range. These waveguide modes give rise to attractive (or repulsive) optical forces between the nanobeams, which in turn affects their mechanical configuration and results in the shift of the optical resonance of the filter [3] , [7] , [21] , [22] . In contrast to previous work [5] , [23] , [24] , [25] , our waveguide-pump approach enables operation using a broadband source in terms of actuation and tuning of the filter resonance. In addition, our devices are fully integrated and fabricated in a technologically relevant silicon-on-insulator (SOI) platform. One drawback of Si, when compared with, for example, Si 3 N 4 (refs 5 , 23 , 24 , 25 ), is significant two-photon absorption that results in heating of the structure and its thermo-optic tuning. In order to elucidate the interplay between OM and thermo-optic effects on the tunability of the silicon-based OM systems, we propose and demonstrate a novel temperature self-referencing approach that takes advantage of higher-order resonances of the structure. Furthermore, slow thermal response time of our device, much slower than OM response time, allows us to explore pure OM effects by operating at high frequencies (higher than thermal cutoff). Design of PCNCs We designed the PCNCs using a deterministic approach [26] , with a hole-to-hole spacing of 360 nm, a nanobeam width of 440 nm and nanobeam separation of 70 nm. A scanning electron microscope image of the final fabricated device is shown in Fig. 1a with the inset showing the released cavity region (for fabrication details see Methods ). This region supports propagating and localized modes with even (TE + ) and odd (TE − ) symmetry. Mode profiles of localized modes are shown in the inset of Fig. 1b . The same figure shows the dispersion of the even (red) and odd (blue) mode as a function of the spacing between the nanobeams. It can be seen that the even mode is highly sensitive to the spacing while the odd mode is not [20] . OM coupling coefficients ( g om ) were calculated to be 96 GHz nm −1 for the even mode, and g om of 0.73 GHz nm −1 for the odd mode (for 70 nm separation), where g om (ref. 1 ) is defined as the change in the resonance frequency due to a change in the separation of the coupled nanobeams. Excellent agreement between the experimental and simulation value justified the use of the theoretically calculated value of g om in our modelling ( Supplementary Fig. S1 ). 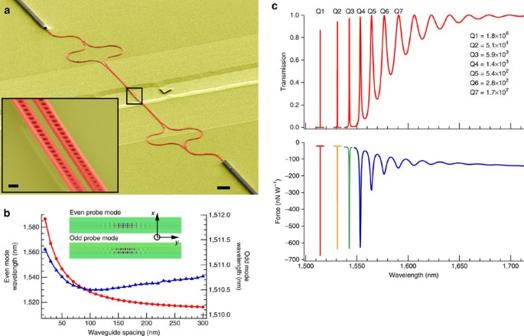Figure 1: Coupled photonic crystal nanobeam cavities. (a) Scanning electron microscope image showing the complete device with the SU-8 coupling pads, balanced Mach–Zehnder interferometer arms, silicon waveguides and the suspended nanobeam cavity region. Scale bar=10 μm. The inset shows the suspended nanocavity in the region given by the black box (inset scale bar=400 nm). (b) The red filled circles and blue filled triangles show the dispersion of the even and odd cavity modes, respectively, for various spacing between the two cavities. The even mode is highly dispersive while the odd mode is not. The device under test had a gap of 70 nm corresponding to an optomechanical coupling coefficient (gom) of 96 GHz nm−1for the even mode and 0.73 GHz nm−1for the odd mode. The inset shows the profiles of the dominant electric field component of the two modes. The cavity modes are localized near the centre of the nanobeams. (c) Simulated transmission of the device for the even electric field profile. The corresponding optical force is in nN W−1generated by the even mode for various pump wavelengths. The negative sign indicates the attractive nature of the force. The force for the first three modes has been rescaled (multiplied by a scaling factor of 1/2,000 (red), 1/60 (yellow) and 1/4 (green)) for better comparison. The transmission spectrum and the mutual optical force between the nanobeams for low-Q modes (Q <104) were calculated using finite-element simulations. The two highest-Q modes with quality factors 1.8×106and 5.1×104were treated using temporal-coupled mode theory. Figure 1c shows a theoretical transmission spectrum of the device under excitation by the even electric field-guided mode, as well as the resulting optical force. One can see that localized cavity modes result in extremely large optical force due to the ultra-high Qs associated with them [1] . This, however, comes at the expense of a very small operational bandwidth. Furthermore, reconfiguration of the filter results in shift of the high-Q cavity resonance, and a wavelength-tracking mechanism is needed ( Supplementary Fig. S2 and Supplementary Discussion ) to keep the pump laser in tune with the structure. This situation, analogous to common gain-bandwidth tradeoff issues in electronics (for example, in amplifiers), can be overcome by taking advantage of broadband waveguide modes [3] supported at the long-wavelength range of our structure, where the optical force is approximately constant over a large wavelength range ( Fig. 1c ). Our structure therefore combines unique advantages of both waveguide-based [3] and cavity-based [1] , [5] , [24] OM systems. One of the unique features of this configuration is that the wavelength of the pump beam can be chosen over a wide wavelength range, so wavelength tracking is not needed to keep the pump in-tune with the structure during the reconfiguration process. Furthermore, broadband light sources ( Supplementary Fig. S3 ) can be used as a pump and the same pump signal can be used to reconfigure a number of filters that operate at different wavelengths (possible applications in filter bank reconfiguration). At the same time, the wavelength scale, high Q, localized modes have excellent sensitivity to mechanical motion, and tuning over several filter linewidths can be achieved using modest pump powers. Therefore, operation at mechanical resonances (which also can require operation in vacuum) is not required [3] . The scheme also allows for independent control of optical and mechanical degrees of freedom (optical and mechanical resonance) of the structure. Finally, an inherent temperature self-referencing scheme can be used to individually evaluate the contributions from thermo-optical and OM effects to the observed detuning in our filters. We do this by taking advantage of cavity modes with odd lateral symmetry, which are in-sensitive to mechanical reconfiguration ( Fig. 1b ) [17] , [20] , but have comparable thermo-optic sensitivities to the even cavity modes (see Methods ). Figure 1: Coupled photonic crystal nanobeam cavities. ( a ) Scanning electron microscope image showing the complete device with the SU-8 coupling pads, balanced Mach–Zehnder interferometer arms, silicon waveguides and the suspended nanobeam cavity region. Scale bar=10 μm. The inset shows the suspended nanocavity in the region given by the black box (inset scale bar=400 nm). ( b ) The red filled circles and blue filled triangles show the dispersion of the even and odd cavity modes, respectively, for various spacing between the two cavities. The even mode is highly dispersive while the odd mode is not. The device under test had a gap of 70 nm corresponding to an optomechanical coupling coefficient ( g om ) of 96 GHz nm −1 for the even mode and 0.73 GHz nm −1 for the odd mode. The inset shows the profiles of the dominant electric field component of the two modes. The cavity modes are localized near the centre of the nanobeams. ( c ) Simulated transmission of the device for the even electric field profile. The corresponding optical force is in nN W −1 generated by the even mode for various pump wavelengths. The negative sign indicates the attractive nature of the force. The force for the first three modes has been rescaled (multiplied by a scaling factor of 1/2,000 (red), 1/60 (yellow) and 1/4 (green)) for better comparison. The transmission spectrum and the mutual optical force between the nanobeams for low-Q modes (Q <10 4 ) were calculated using finite-element simulations. The two highest-Q modes with quality factors 1.8×10 6 and 5.1×10 4 were treated using temporal-coupled mode theory. Full size image Experimental setup The devices were probed using a butt coupling technique using two lensed fibres ( Supplementary Fig. S4 and Methods ). Unlike tapered fibre [27] probing, this type of characterization method remains invariant under any mechanical oscillations of the suspended waveguides and can be easily integrated for on-chip applications. Light from a tunable laser was amplified using an erbium-doped fibre amplifier (EDFA) and used as the pump while another tunable laser was used to probe the structure. A schematic of the experimental setup is shown in Fig. 2a . 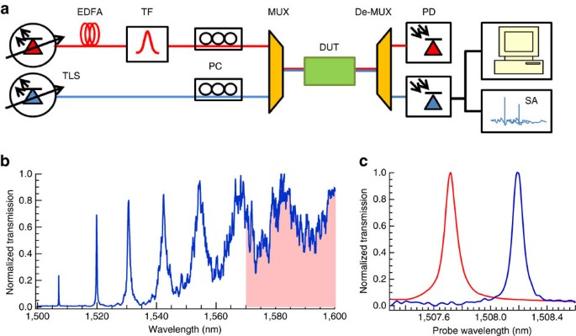Figure 2: Experimental results for waveguide-pump–cavity-probe system. (a) Schematic diagram of the pump-probe characterization setup used in the experiment. The cavity resonance was probed using a tunable laser (Santec TLS 510) and a fast, sensitive InGaAs detector (New Focus). Another tunable laser was used as the pump and was amplified using a high-power output EDFA (L Band Manlight). The input and output WDM (wavelength division multiplexer; MicroOptics) ports were designed to operate in the 1,470–1,565 nm and 1,570–1,680 nm ranges. The mechanical response of the devices was studied using a real-time spectrum analyser (Tektronix RSA 3300). De-MUX, de-multiplexer; DUT; device under test; EDFA, erbium-doped fibre amplifier; MUX, multiplexer; PC, polarization controller; PD, photo detector; SA, spectrum analyser; TF: tunable filter; TLS, tunable laser source. (b) A transmission spectrum of the fabricated cavity. The transmission has been normalized to the maximum value outside the bandgap. The fundamental even mode is found to be near 1,507 nm with a Q of 15,000. The shaded region shows the operating range of the EDFA used to amplify the pump. The pump has a waveguide-like mode profile (seeSupplementary Fig. S6) as it is outside the bandgap and is used to induce mechanical deformation to detune the even mode cavity resonance. (c) Cavity resonance was tuned from 1,507.72 to 1,508.19 nm when 6 mW of pump power at 1,583 nm was used. Red and blue curves correspond to 0 and 6 mW of pump power. The transmission in this case has been normalized to the maximum value of the cavity resonance. Cavity tuning was due to contribution from thermo-optical, nonlinear optical and optomechanical effects. Figure 2: Experimental results for waveguide-pump–cavity-probe system. ( a ) Schematic diagram of the pump-probe characterization setup used in the experiment. The cavity resonance was probed using a tunable laser (Santec TLS 510) and a fast, sensitive InGaAs detector (New Focus). Another tunable laser was used as the pump and was amplified using a high-power output EDFA (L Band Manlight). The input and output WDM (wavelength division multiplexer; MicroOptics) ports were designed to operate in the 1,470–1,565 nm and 1,570–1,680 nm ranges. The mechanical response of the devices was studied using a real-time spectrum analyser (Tektronix RSA 3300). De-MUX, de-multiplexer; DUT; device under test; EDFA, erbium-doped fibre amplifier; MUX, multiplexer; PC, polarization controller; PD, photo detector; SA, spectrum analyser; TF: tunable filter; TLS, tunable laser source. ( b ) A transmission spectrum of the fabricated cavity. The transmission has been normalized to the maximum value outside the bandgap. The fundamental even mode is found to be near 1,507 nm with a Q of 15,000. The shaded region shows the operating range of the EDFA used to amplify the pump. The pump has a waveguide-like mode profile (see Supplementary Fig. S6 ) as it is outside the bandgap and is used to induce mechanical deformation to detune the even mode cavity resonance. ( c ) Cavity resonance was tuned from 1,507.72 to 1,508.19 nm when 6 mW of pump power at 1,583 nm was used. Red and blue curves correspond to 0 and 6 mW of pump power. The transmission in this case has been normalized to the maximum value of the cavity resonance. Cavity tuning was due to contribution from thermo-optical, nonlinear optical and optomechanical effects. Full size image A measured transmission spectrum of the device (similar to the one shown in Fig. 1a ) is shown in Fig. 2b with the fundamental even mode at 1,507.72 nm (the slight discrepancy in the measured and simulated resonance wavelength shown in Fig. 1c is due to the error associated in measuring the dimensions using a scanning electron microscope image). The shaded portion under the transmission curve denotes the pump region, which lies outside the bandgap of the photonic crystal. We note that due to the limited tuning range of the pump EDFA, in our experiments, the pump is not positioned in the flat part of the transmission spectrum. Therefore, the pump benefits from the light confinement and low-Qs of extended resonances of the structure (broad peaks in the transmission spectrum). Based on theoretical predictions, we estimate that the force associated with this effect is approximately twice as big as the force in the flat part of the spectrum ( Fig. 1c ). When the pump laser excites only the even mode, an attractive optical force is generated, which reduces the separation between nanobeams and red-detunes the even probe mode. Figure 2c shows the experimental detuning of the fundamental even mode with a 6 mW pump (estimated power inside the waveguide just before the photonic crystal) at 1,583 nm. This detuning is in part due to OM effects, and in part due to the combination of thermo-optic (Th), free carrier dispersion (FCD) and Kerr effects. The overall detuning of the modes is given by: We theoretically estimated the contributions of these nonlinear effects ( Supplementary Fig. S5 ) and found that in addition to OM detuning, thermo-optic effects play an important role in the detuning of the cavity resonance (both even and odd modes shift towards longer wavelengths with increasing temperature). For the given input power range, themo-optic effects can be as high as 80% ( Supplementary Methods ). However, due to the nonlinear dependence of thermo-optic effect on pump power, its contribution increases at higher powers, whereas the OM effect remains linear. Decoupling thermo-optic and OM effects In order to decouple thermal and mechanical effects, we used an odd-localized mode ( Supplementary Fig. S6 ) of the cavity as an on-chip temperature reference. This is possible as this mode's resonance does not tune with mechanical motion ( Fig. 1b ), and tunes only with temperature. The experimentally determined ratio of the temperature shifts of the even and odd mode is 0.93 (see Methods ), and is due to slightly different overlaps of the two modes with the silicon nanobeams. In order to simultaneously excite the even and the odd probe modes, and use the odd cavity mode as a built-in temperature reference, we incorporated an unbalanced Mach–Zehnder interferometer (MZI) before the cavities ( Supplementary Fig. S7 ). This scheme is also useful to actuate the device using odd pump mode and generate repulsive force. However, as can be seen from Fig. 1b , the dispersion for the odd mode is extremely small. As a result, the g om for the odd mode is about two orders of magnitude smaller when compared with the even mode. This holds true even for the odd low-Q waveguide-like modes used as the pump (checked using numerical modelling). Therefore, in our system, repulsive force resulting from the odd pump modes is orders of magnitude smaller than the attractive force induced by the even mode. It is interesting to note that the dispersion of the localized odd cavity mode (probe) switches sign at about 110 nm of separation between nanobeams. Below this gap, the force generated by the odd probe mode is attractive while it is repulsive for larger gaps. However, the force is extremely small (especially for larger gaps) and is not detectable in the current setup with the available pump power levels: we calculated the expected tuning due to the localized odd cavity mode to be about 20 times smaller in our devices with 70 nm separation. 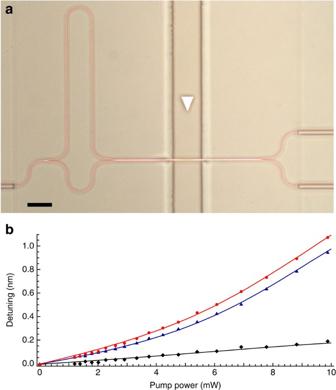Figure 3: Evaluation of optomechanical effect using temperature self-referencing. (a) Optical micrograph of a device with an unbalanced MZI for simultaneous measurement of both the even and odd modes. Scale bar=20 μm. (b) Tuning of the cavity resonance for various pump powers and fixed pump wavelength of 1,573.5 nm. The red circles and blue triangles correspond to even and odd modes, whereas the black diamonds show the optomechanical detuning of the even mode. The latter was obtained by first determining the ratio of detuning for the even and odd modes due to purely thermal effects, by heating the sample (seeMethods). As the odd mode was sensitive only to temperature, it was used as a temperature sensor and the even mode temperature detuning was estimated using the above ratio and subtracted from the total detuning of the even mode. Using this self-referencing technique, we estimated that more than 20% of the total tuning is due to purely optomechanical effects. Solid lines refer to the expected detunings. Figure 3a shows an optical micrograph of the new configuration. In this case, the cavity resonance (even mode) was at 1,524.9 nm. Figure 3b shows the experimentally measured detuning of the probe modes (even and odd) for various pump powers (estimated power inside the waveguide just before the photonic crystal) and pump wavelength of 1,573.5 nm. The change in the resonances of both the even and odd modes are denoted with red circles and blue triangles, respectively, whereas the shift resulting solely from the OM effect is shown with black diamonds. The latter was obtained as proportional difference of the shifts of even and odd modes. The solid lines in Fig. 3b were obtained using equation (1). Thermal, FCD, Kerr and OM contributions of the pump and probe along with the cross coupling terms were included. The change in stored energy due to self-detuning of the pump was also computed and included in the estimation ( Supplementary Methods ). The significance of thermo-optic effects is clearly seen, and 80% of tuning is attributed to this effect. Therefore, in contrast to Si 3 N 4 -based OM structures, Si-based ones do suffer from significant two-photon absorption-induced thermo-optic effects. Figure 3: Evaluation of optomechanical effect using temperature self-referencing. ( a ) Optical micrograph of a device with an unbalanced MZI for simultaneous measurement of both the even and odd modes. Scale bar=20 μm. ( b ) Tuning of the cavity resonance for various pump powers and fixed pump wavelength of 1,573.5 nm. The red circles and blue triangles correspond to even and odd modes, whereas the black diamonds show the optomechanical detuning of the even mode. The latter was obtained by first determining the ratio of detuning for the even and odd modes due to purely thermal effects, by heating the sample (see Methods ). As the odd mode was sensitive only to temperature, it was used as a temperature sensor and the even mode temperature detuning was estimated using the above ratio and subtracted from the total detuning of the even mode. Using this self-referencing technique, we estimated that more than 20% of the total tuning is due to purely optomechanical effects. Solid lines refer to the expected detunings. Full size image Pulsed operation One way of reducing the relative contribution of thermo-optical effects in our devices is to improve g om by using nanobeams with smaller gaps. This, however, is challenging with our current fabrication capabilities. Another method is to excite the structure with modulated pump beam with repetition rates faster than the thermal response (measured value: 100 kHz) but lower than the mechanical resonance of the structure (measured: 6.7 MHz). In this way, the structure would 'thermalize' and would not be able to respond to changes in temperature, and the OM effects would remain as the dominant tuning mechanism. Importantly, such dynamic, modulated, operation closely resembles the situation found in practices, including optical circuit switching and optical burst switching, where optical circuits are reconfigured with frequencies typically larger than our thermal cutoff frequency. Thermal cutoff and mechanical resonance frequencies define three distinct operating regimes of our structure ( Fig. 4 and see Methods ). In Region 1, operating frequency is below the thermal cutoff frequency and both thermo-optical and OM effects can follow the modulation resulting in resonance tuning over wide wavelength range. In Region 2, the operating frequency is larger than the thermal cutoff frequency but smaller than mechanical resonance and the response is entirely due to OM effects. The wavelength tuning is smaller in this region than in Region 1, which is consistent with our observations that at low frequencies thermal effects cause roughly four times more tuning than mechanical ones. Still, this tuning range is suitable for optical switching applications where it is sufficient to detune the cavity resonance off the wavelength of the optical data signal. Fig. 4b shows the normalized line scans in Regions 2 and 3 proving the existence of OM effect for the even mode in Region 2 and the absence of any thermo-optical effect in either of the regions (as seen from the corresponding line scans for the odd mode). We note that, as expected at mechanical resonance, the tuning range of the even mode is large, as the nanobeam motion is amplified by the mechanical Q (Q mech ~17). Finally, in Region 3 the operating frequency is larger than mechanical cutoff frequency, and neither thermal nor OM effects can keep up with the modulation, resulting in negligible tuning. 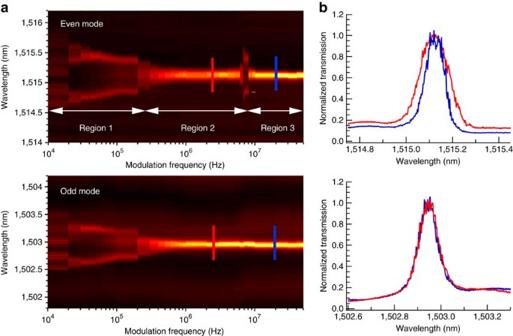Figure 4: Detuning of the even and odd modes for pulsed pump operation. (a) Three regions of operation, defined by the thermal cutoff and mechanical cutoff frequencies, can be identified. Region 1 denotes the regime where thermo-optic and optomechanical effects are prominent, as structure can respond both thermally and mechanically to the modulation signal. This regime extends from dc operation to thermal cutoff frequency. Here cavity resonance is modulated over a wide wavelength range, due to a combination of thermal and mechanical effects, and it appears smeared-out by the slow detector used (seeMethods). Region 2 denotes the regime above the thermal cutoff frequency, where thermal effects settle to a steady state value and only the optomechanical effects are prominent. This regime extends from the thermal cutoff to mechanical cutoff frequency. This is precisely the regime where optomechanics is the dominant tuning mechanism. The wavelength smearing is smaller in this region than in Region 1, which is consistent with our observations that thermal effects cause roughly four times more tuning than mechanical effects in the case of dc actuation. Also, as expected there is no smearing in the odd-mode resonance in this regime as itsgomis very low. Region 3 denotes the regime above the mechanical cutoff frequency, where both the thermo-optic and optomechanical effects are too slow to follow the modulation signal. The high detuning in the even mode at the mechanical frequency (~6.7 MHz) is due to enhancement of the motion because of mechanical Q but is absent in the case of the odd mode due to its lowgom. (b) Normalized (to the maximum value of the individual resonance) line scans for even and odd cavity mode detunings in Regions 2 and 3. The red and blue curves correspond to red and blue lines drawn ina. Smearing is observed for the even mode while it is absent for the odd mode, showing the prominence of optomechanical effect in Region 2. Figure 4: Detuning of the even and odd modes for pulsed pump operation. ( a ) Three regions of operation, defined by the thermal cutoff and mechanical cutoff frequencies, can be identified. Region 1 denotes the regime where thermo-optic and optomechanical effects are prominent, as structure can respond both thermally and mechanically to the modulation signal. This regime extends from dc operation to thermal cutoff frequency. Here cavity resonance is modulated over a wide wavelength range, due to a combination of thermal and mechanical effects, and it appears smeared-out by the slow detector used (see Methods ). Region 2 denotes the regime above the thermal cutoff frequency, where thermal effects settle to a steady state value and only the optomechanical effects are prominent. This regime extends from the thermal cutoff to mechanical cutoff frequency. This is precisely the regime where optomechanics is the dominant tuning mechanism. The wavelength smearing is smaller in this region than in Region 1, which is consistent with our observations that thermal effects cause roughly four times more tuning than mechanical effects in the case of dc actuation. Also, as expected there is no smearing in the odd-mode resonance in this regime as its g om is very low. Region 3 denotes the regime above the mechanical cutoff frequency, where both the thermo-optic and optomechanical effects are too slow to follow the modulation signal. The high detuning in the even mode at the mechanical frequency (~6.7 MHz) is due to enhancement of the motion because of mechanical Q but is absent in the case of the odd mode due to its low g om . ( b ) Normalized (to the maximum value of the individual resonance) line scans for even and odd cavity mode detunings in Regions 2 and 3. The red and blue curves correspond to red and blue lines drawn in a . Smearing is observed for the even mode while it is absent for the odd mode, showing the prominence of optomechanical effect in Region 2. Full size image Dynamical OM effects We characterized the Brownian motion of the two nanobeam cavities, in ambient conditions, by detuning the probe to the maximum slope of the cavity resonance (point A in Fig. 5a inset). As the even mode of the coupled cavity system is extremely dispersive with respect to the gap between the beams, any motion of the beams is transduced onto the transmission of the cavity. This modulated transmission of the probe was analysed using a spectrum analyser and is shown in Fig. 5a . Various in-plane and out-of-plane vibrational modes can be identified in the spectrum ( Supplementary Fig. S8 ). The fundamental in-plane mode, which has the maximum g om , shows up as a very strong peak at 8 MHz. The second and third order in-plane modes can also be well resolved in the spectrum. We note that the peak at 16 MHz does not correspond to any vibrational mode and is an artefact of nonlinear transduction (see Supplementary Fig. S9 and Supplementary Discussion ). 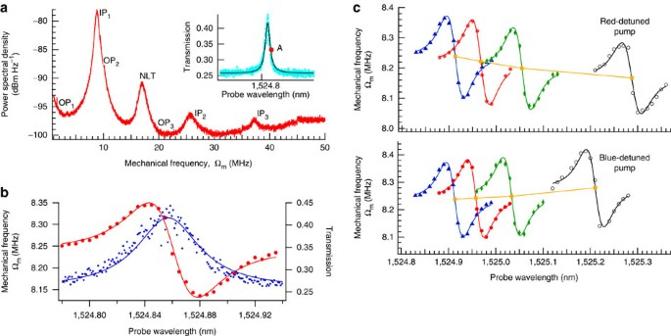Figure 5: Dynamic optomechanical effects. (a) Noise spectrum showing the Brownian motion of the coupled PCNCs. The power spectral density spectrum shows the various mechanical modes of the nanobeams. The peaks are labelled according to their mechanical deflection, which can be in-plane (IP) or out-of-plane (OP). The inset shows the optical spectrum with operating point (point A), corresponding to the maximum slope of the transmission resonance, indicated. The most efficient transduction is obtained for fundamental in-plane mode IP1(Supplementary Fig. S8). The peak at 16 MHz does not correspond to any mechanical mode, but is a Fourier component due to nonlinear transduction (NLT). This happens when Brownian motion of the beams is large enough to detune the probe laser across the Lorentzian line shape of the cavity resonance (Supplementary Fig. S9andSupplementary Discussion). In this case, the relation between optical transmission and gap is no longer linear around the operating point A. The measured electrical noise floor was −103 dBm Hz−1near 10 MHz. (b) Mechanical response of the fundamental in-plane mechanical mode IP1(red circles) for various detuning of the probe mode (blue dots) at zero pump power. This effect is due to self-stiffening of the nanobeams due to large optical energy stored inside the cavities. The solid red line is the fit given by equation (2) and the solid blue line is a Lorentzian fit for the optical mode. (c) The shift in mechanical response shown inbfor various pump power at two different pump detunings. The red-detuned pump was set at 1,570.5 nm, while the blue-detuned pump was set at 1,573.5 nm. The mechanical response moves towards lower frequencies for red detuning and towards higher frequencies for a blue-detuned pump. The blue triangles, red circles, green diamonds and the unfilled black circles correspond to 0, 0.75, 1.6 and 3.3 mW of pump power, respectively, and the corresponding solid lines are the fits given by equation (2). The yellow squares represent the mechanical frequency of the probe without self-stiffening from the probe. The yellow line is a guide to the eye. Figure 5b plots the effect of probe detuning on the resonant frequency of the fundamental, mechanical, in-plane mode. The blue curve shows the optical transmission spectrum of the even mode, whereas the red curve plots the detuning of the mechanical resonance for various probe detuning. As the device operates in the sideband unresolved limit (Ω M ≪ optical Q ), the response is only due to optical stiffening [1] ( Supplementary Fig. S10 ) and is given by: Figure 5: Dynamic optomechanical effects. ( a ) Noise spectrum showing the Brownian motion of the coupled PCNCs. The power spectral density spectrum shows the various mechanical modes of the nanobeams. The peaks are labelled according to their mechanical deflection, which can be in-plane (IP) or out-of-plane (OP). The inset shows the optical spectrum with operating point (point A), corresponding to the maximum slope of the transmission resonance, indicated. The most efficient transduction is obtained for fundamental in-plane mode IP 1 ( Supplementary Fig. S8 ). The peak at 16 MHz does not correspond to any mechanical mode, but is a Fourier component due to nonlinear transduction (NLT). This happens when Brownian motion of the beams is large enough to detune the probe laser across the Lorentzian line shape of the cavity resonance ( Supplementary Fig. S9 and Supplementary Discussion ). In this case, the relation between optical transmission and gap is no longer linear around the operating point A. The measured electrical noise floor was −103 dBm Hz −1 near 10 MHz. ( b ) Mechanical response of the fundamental in-plane mechanical mode IP 1 (red circles) for various detuning of the probe mode (blue dots) at zero pump power. This effect is due to self-stiffening of the nanobeams due to large optical energy stored inside the cavities. The solid red line is the fit given by equation (2) and the solid blue line is a Lorentzian fit for the optical mode. ( c ) The shift in mechanical response shown in b for various pump power at two different pump detunings. The red-detuned pump was set at 1,570.5 nm, while the blue-detuned pump was set at 1,573.5 nm. The mechanical response moves towards lower frequencies for red detuning and towards higher frequencies for a blue-detuned pump. The blue triangles, red circles, green diamonds and the unfilled black circles correspond to 0, 0.75, 1.6 and 3.3 mW of pump power, respectively, and the corresponding solid lines are the fits given by equation (2). The yellow squares represent the mechanical frequency of the probe without self-stiffening from the probe. The yellow line is a guide to the eye. Full size image where where Ω M is the mechanical eigenfrequency, g om is the OM coupling constant, m eff is the effective mass of the mechanical mode, Δ′ c,p are the detuning of the input laser, | a c,p | 2 are the energies stored in the respective modes and Γ′ c,p is the decay rate of the stored energy in the optical modes. Apart from the self-stiffening effect due to the probe mode as seen in Fig. 5b , stiffening can also be induced by the pump. This effect is studied by pumping at either side of the broad pump mode. As the power in the pump mode is increased the mechanical resonance of the device is detuned due to stiffening. The sign of this mechanical resonance detuning is dependent on the detuning of the pump laser with respect to the pump resonance ( Fig. 5c ). For a red-detuned pump the beams are softened and the mechanical resonance frequency decreases, whereas blue detuning results in an increase of the mechanical frequency. The smooth curves show the fits using equation (2) taking into account the presence of the pump. Therefore, our approach allows us to independently control the optical and mechanical frequencies of our OM filters. We note that in addition to attractive forces discussed above, repulsive force can also be obtained by exciting odd pump modes. This force, however, is much weaker due to small g om of the odd mode in our structure and does not result in observable effects. Our devices are fully integrated and made in technologically relevant SOI platform. This comes at an expense of significant two-photon absorption-induced thermo-optic effects. Using an on-chip temperature-sensing scheme, we successfully elucidate the interplay between OM and thermo-optic effects on the tunability of the silicon-based OM filters. We demonstrated that OM effects dominate the thermal ones when structure is operated at frequencies higher than its thermal cutoff frequency. This is of practical importance for applications in all-optical circuit switching and packet routing. Furthermore, for these applications it is sufficient to detune the resonance of the cavity for few linewidths only in order to get it off resonance with incoming optical signal. In conclusion, we demonstrated an all-optical tunable filter using coupled photonic crystal nanobeam cavities, where a considerable portion of the tuning is affected by mechanical reconfiguration. Specifically, we measured a total tuning of filter resonance of more than 18 linewidths, out of which 20% was due to OM effects. As demonstrated, OM-tuning effects are much faster than the thermal ones in our system, which is important for practical applications. The operating speed of OM devices could be pushed into the gigahertz regime by using smaller and stiffer structures, at the expense of the increased optical power needed to actuate them. Our scheme allows for a wide range of pump wavelength selection while overcoming the limitation of self-detuning of the pump and can be used to simultaneously control multiple devices. At the same time, independent control over the mechanical response was also achieved by varying the pump laser's wavelength. Our technique is a promising candidate for realization of reconfigurable and programmable optical devices, including filters and filter banks, routers and modulators. Device fabrication and characterization The devices were fabricated on a SOI substrate with a silicon device layer of 220 nm and a buried oxide layer of 3 μm. The width and thickness of each nanobeam was 440 and 220 nm, respectively, whereas the periodicity of the holes was 360 nm. The separation between the beams was 70 nm. The patterns were written using conventional 100 keV e-beam lithography using negative e-beam resist XR-1451-002 (hydrogen silsesquioxane) and transferred to the device layer using inductively coupled plasma reactive-ion etching (ICP-RIE) with a chlorine-based chemistry. Proximity correction was necessary in order to achieve correct hole sizes for narrow waveguide gaps. In the second fabrication step, SU-8 polymer coupling pads were fabricated on each end of the device to couple light on and off the chip. After this step, Shipley 1813S photoresist was spun on the sample. The area excluding the SU-8 pads was exposed using photolithography. The remaining e-beam resist covering the waveguides was removed by dipping the sample in 7:1 buffered oxide etch (BOE) for 1 min. The sample was then cleaved through the SU-8 pads and another photolithography step was carried out to open a small window in order to suspend the PCNCs. Finally, the cavities were under-etched using 7:1 BOE and then dried in a critical point dryer. The etch time was adjusted to achieve an etch depth of 2 μm. A pump-probe scheme was used to test the devices as shown in Fig. 1b . Light was coupled using polarization maintaining (PM)-tapered lensed fibre (Oz optics, NA 0:4) into the SU-8 waveguide ( Supplementary Fig. S4a ). An inverse taper geometry [28] was used as a spot-size converter to efficiently transfer the light from SU-8 waveguides into the silicon waveguides. This was necessary because SU-8 waveguides has significantly larger dimensions (3×3 μm 2 ) when compared with silicon waveguides (440×220 nm 2 ). At the output, a similar coupling method was used except the light was collected with a single mode (SM)-tapered lensed fibre ( Supplementary Fig. S4b ; SM-tapered fibres have lower taper conversion loss). The propagation loss of the silicon waveguides and the maximum bend loss for 10 μm bend radius were measured to be 4.5 dB cm −1 and 1.0 dB, respectively. This was measured by imaging the light scattered from the waveguide from top with a sensitive infrared camera. The SU-8 waveguide propagation loss was measured with the same method and found to be 7 dB cm −1 . This is likely due to the excitation of higher-order modes of the SU-8 waveguides that are less confined and prone to higher losses. By measuring the insertion loss for the waveguide samples and using the measured propagation losses of the waveguides, we estimated the coupling loss associated with the spot-size converters to be 2±0.5 dB. This was further confirmed by reversing the input signal direction. The power in the waveguide just before the cavity was estimated using the above-measured values of coupling and propagation losses and the known device dimensions. The energy stored inside the cavity ( W ) is determined by taking into account the total Q (Q t ) and the waveguide coupling Q (Q c ) for the particular mode: W =4Q t 2 P in /( ω 0 Q c ). Unless otherwise stated, the power throughout the manuscript is the estimated value inside the waveguide just before the photonic crystal. The devices were characterized using tunable lasers (Agilent 81682, Agilent Techmologies; Santec TSL-510, Santec) and a sensitive InGaAs detector (EO systems, IGA-010-TE2-H). For mechanical measurements, a fast InGaAs detector (Newport, 1811-FC) was used along with an external amplifier (Stanford Research Systems) before analysing the signal using an electrical spectrum analyser (Tektronix, RSA3003). The pump laser signal was amplified using an L band 1 W EDFA (Manlight). The EDFA output was filtered for ASE emissions using a tunable filter (Agiltron). The pump and probe signals were multiplexed and de-multiplexed using a wavelength-division multiplexing (MicroOptics). Thermal tuning and calibration of the even and odd modes Silicon has a relatively large thermo-optic coefficient, d n Si /d T =1.86×10 −4 K −1 . As a result, any change in temperature modifies the resonance frequency of the cavity ( Supplementary Methods , equations S29–S31). This temperature detuning is slightly different for each mode because of different mode overlap factors with silicon ( Supplementary Methods , equations S29–S31). Hence, it is important to characterize the tuning due to temperature for each mode, especially for the mode used for on-chip temperature calibration. This was determined experimentally by measuring the resonance frequency of both the even and odd modes as a function of temperature. The sample was placed on a thermo-electric heater and the temperature on the sample surface was measured. The ratio of wavelength detuning with temperature of the two modes was determined from the slope of the temperature versus detuning curves. The experimentally determined value of tuning ratio of the even mode to the odd mode was found to be 0.93. This value was used in all the calculations. Excitation using an unbalanced MZI We considered only TE-polarized modes throughout this work. Our devices support both highly localized cavity modes with large Q-factors and extended waveguide-like modes with low Q-factors. Because of the symmetry of the structure with respect to mirror plane in the middle of the gap (perpendicular to the substrate), both localized and extended modes have either even or odd symmetry ( Supplementary Fig. S6 ). The high-Q modes were considered as probe/filter and low-Q modes were used to pump and actuate the devices. We aimed to tune the resonance frequency of the filter modes by using OM actuation when the devices were excited with a low-Q pump mode. To excite the even and odd modes simultaneously, we incorporated an unbalanced MZI at the input of the device (200 μm path difference). An unbalanced MZI generates a phase difference between its output arms. This phase difference depends on the wavelength and the difference between the lengths of the MZI arms. When the phase difference is 0, the even mode is excited, and when the phase is π the odd mode is excited. For phase difference in the range between 0 and π , both even and odd modes are excited. The signal at the output (after the cavities) from each of the waveguides was collected without combining them. This allowed us to excite and collect both even and odd modes of the structure ( Supplementary Fig. S7 ). For the experimental results shown in Fig. 2 , we decided to use a balanced MZI to split the power equally in the two waveguides instead of redesigning a 3-dB coupler. Reduced thermal effects by pulsed excitation Figure 4 shows the results of the experiment when the control beam was modulated by using an electro-optical modulator (a modulation depth of ~40% was used, which was limited by the modulator). A 50% duty cycle square wave was applied using a signal generator. The response of the even and odd filter modes were characterized with a tunable laser and a sensitive but slow detector (1 kHz bandwidth). The slow detector was particularly useful in capturing the tuning of the resonances for modulation frequencies higher than 1 kHz: for modulation frequencies higher than 1 kHz, the optical signal on the detector changed faster than the response time of the detector (or the cavity resonance was detuned at a rate much faster than the response time of the detector), and the detector averaged out all fluctuations and generated a cleaner signal. We also note that the laser was scanned at a speed of 5 pm ms −1 , and therefore the detector produced an averaged output of the optical signal for every 5 pm of cavity detuning. How to cite this article: Deotare, P. B. et al . All optical reconfiguration of optomechanical filters. Nat. Commun. 3:846 doi: 10.1038/ncomms1830 (2012).